Nacre-mimetics with synthetic nanoclays up to ultrahigh aspect ratios Nacre-mimetics hold great promise as mechanical high-performance and functional materials. Here we demonstrate large progress of mechanical and functional properties of self-assembled polymer/nanoclay nacre-mimetics by using synthetic nanoclays with aspect ratios covering three orders in magnitude (25–3,500). We establish comprehensive relationships among structure formation, nanostructuration, deformation mechanisms and mechanical properties as a function of nanoclay aspect ratio, and by tuning the viscoelastic properties of the soft phase via hydration. Highly ordered, large-scale nacre-mimetics are obtained even for low aspect ratio nanoplatelets and show pronounced inelastic deformation with very high toughness, while those formed by ultralarge nanoplatelets exhibit superb stiffness and strength, previously only reachable for highly crosslinked materials. Regarding functionalities, we report formerly impossible glass-like transparency, and excellent gas barrier considerably exceeding earlier nacre-mimetics based on natural nanoclay. Our study enables rational design of future high-performance nacre-mimetic materials and opens avenues for ecofriendly, transparent, self-standing and strong advanced barrier materials. The excellent mechanical performance of biological materials originates from a hierarchically ordered arrangement of well-tailored hard and soft building blocks [1] , [2] , [3] . The hard matter serves as the load bearing and reinforcing part, whereas energy can be dissipated into the soft segments. As a direct consequence, many of these materials combine high toughness with excellent strength and stiffness. For instance, in nacre, the layered arrangement of platelet-shaped CaCO 3 crystals and biopolymers in a brick-and-mortar structure leads to a synergistic mechanical performance [4] . The Young’s modulus can reach up to 40–70 GPa, ultimate tensile strength is as high as 80–135 MPa and the toughness is 3,000 times higher than that of an aragonite monolith [4] , [5] , [6] , [7] . Considering the lightweight character of mechanically strong and tough biomaterials, finding corresponding biomimetic materials that allow large-scale and facile preparation for future load-bearing applications is of preeminent importance [8] . For nacre-mimetics, highly ordered, layered nanocomposite structures with high level of reinforcements, and with tailored interfaces and preferentially tailored molecular energy dissipation mechanisms are being pursued. However, this is a major scientific and technological challenge as precise nanostructuration at such biomimetic compositions with high fractions of reinforcements is hard to combine with large-scale processing methods. Various efforts have been undertaken to mimic the layered hard/soft composite structure of nacre [9] via for example, several sequential approaches, such as LbL [10] , [11] , [12] , [13] , [14] , [15] , [16] , [17] , [18] and other multilayer deposition strategies [19] , [20] , ice-templating and sintering of ceramics [21] , [22] , [23] , spray coating [24] , [25] , glow discharge plasma deposition [26] , uncontrolled co-casting of polymer/clay mixtures [27] , [28] , or processes at interfaces [29] , [30] . Unfortunately, many of these approaches are limited to a very small scale, and remain technologically infeasible owing to energy-intensive and laborious multistep procedures. Moreover, considering the needs in the application world, we also have to identify further possibilities arising from the excellent nanostructural control. The goal is to expand the property profiles beyond pure mechanical performance and implement new concepts for multifunctional biomimetic materials, highly relevant for future technologies. Such properties include fire and gas barrier properties, anisotropic thermal, electric or ionic conductivity, while at the same time possibly reaching glass-like transparency and maintaining excellent mechanical properties. Two dimensional (2D) clay nanosheets are among the most interesting building blocks to realize these outstanding challenges owing to their high interface, nanoscale dimensions and tunable aspect ratio. Previous reports mostly concentrated on individual functional properties, such as gas barrier [27] , [31] , [32] , [33] , [34] , [35] , [36] , [37] , fire shields [35] , [36] , [37] , [38] , [39] and photothermal activity [25] while still often falling short of addressing and realizing multifunctional property profiles with best and optimized performance in different areas. Recently Walther et al. [36] introduced a fast, facile and scalable concept to achieve superb control over nanostructuration in nacre-mimetics via self-assembly of core/shell nanoplatelets formed by adsorption of soft polymers onto hard nanoclays. The resulting core/shell nanoplatelets undergo concentration-induced self-assembly on a macroscopic-length scale during water removal owing to the excluded volume effects. Such self-assembled artificial nacre is characterized by maximum exfoliation and at the same time maximum amount of inorganic reinforcements arranged in a highly ordered fashion. The polymer shell pre-encodes the properties of the soft energy-dissipating layer on the reinforcing nanoplatelets. Recent studies shed light on how polymer dynamics and supramolecular binding scenarios within the soft phase influence the macroscopic mechanical properties, and how sacrificial bonds and synergetic mechanical performance can be targeted based on controlling the molecular interactions [40] , [41] , [42] , [43] . The overall process is environmentally friendly and economic. We further simplified the method to a direct mixing approach of highly concentrated dispersions (>10 wt%) using suitably tailored nanoclay and polymer [44] . However, much in contrast to previous work on understanding and evolving the soft phase [42] , [45] , very little is known about the possibilities arising from changing the nanoclay. Research on clay-based nacre-mimetics has so far almost exclusively focused on using montmorillonite (MTM), a natural bentonite clay that mostly exfoliates into 1 nm thick clay sheets with an average diameter of a few hundred nanometres in water. MTM, however suffers from major drawbacks. First of all, its aspect ratio cannot be tuned. This is however of profound importance for an in-depth understanding of the mechanical properties of such advanced, nanostructured composites with nanoconfined polymer layers and subtle nanomechanics. In addition, the optical quality is poor because natural MTM is contaminated by iron or other metal ions and their corresponding oxides leading to a yellowish colour. Furthermore, the non-perfect surface charge distribution and presence of fractions of larger agglomerates can lead to imperfect exfoliation and contamination with unwanted larger particles, requiring fractionation steps and leaving ambiguities in determining clear structure/property relationships [46] , [47] . All these factors, absorption due to contamination, light scattering because of larger particles and non-complete exfoliation inevitably lead to coloured and at best only translucent films once a certain thickness is reached. Here we demonstrate distinct advantages of using synthetic nanoclays with widely different aspect ratios up to 10,000 for self-assembled artificial nacre based on polyvinylalcohol (PVA)-coated nanoclay. Such synthetic nanoclays are free from colour contamination, unlike natural clays, possess homogeneous charge distribution on the surface and fully exfoliate into single nanosheets in water. We establish the relationships among structure formation, nanostructuration, deformation mechanisms and mechanical properties as a function of aspect ratio and also by tuning the viscoelastic properties of the soft phase through exposure to different levels of hydration. We show that nanocomposites reinforced with low aspect ratio nanoclay have superior toughness owing to pronounced inelastic deformation via platelet pull-out. On the contrary, nacre-mimetics formed by ultralarge synthetic nanoclay open avenues to superb stiffness up to 40 GPa and tensile strength exceeding 200 MPa, thereby attaining elastic properties previously only being in reach after tedious post-crosslinking. We further correlate how the amount of polymer in differently sized clays (very small versus very large ones) influences the transition towards inelastic deformation and stable crack propagation. Excellent gas barrier properties and glass-like transparency complement the scope of mechanical properties and provide design principles for using synthetic nanoclays for multifunctional biomimetics materials as, for example, needed for flexible, advanced barrier materials. Strategy and building blocks and structural characterization The general strategy for the preparation of self-assembled artificial nacre is outlined in Fig. 1a . It is based on the concept that polymer-coated core/shell colloidal-scale nanoplatelets self-assemble into highly ordered lamellar films upon water removal owing to excluded volume effects. These core/shell nanoplatelets are simply prepared by adsorption of specifically binding polymers onto fully exfoliated synthetic nanoclays in aqueous dispersion, followed by removal of excess polymer. This yields very well-defined core/shell particles without excess of polymer and allows to approach highly ordered nacre-mimetics with fully exfoliated synthetic nanoclays at biomimetic compositions. We use PVA because of its known affinity to nanoclays and also because a comparison can be made to earlier nacre-mimetics, either prepared by the layer-by-layer technique or via self-assembly [10] , [15] , [36] , [40] , [45] . 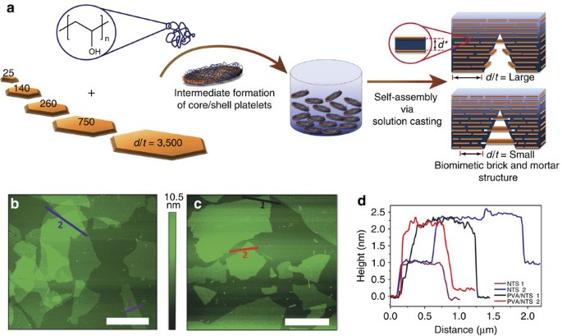Figure 1: Preparation of artificial nacre and AFM characterization of NTS nanoclay before and after coating with PVA. (a) Artificial nacre via concentration-induced self-assembly of polymer-coated nanoclay platelets with intrinsic hard/soft architecture. Well-defined core/shell particles are isolated by centrifugation and redispersion. Different aspect ratios are indicated as diameter to thickness (d/t) and corresponding fracture modes are displayed to the right as influenced by the aspect ratio and polymer content. (b,c) AFM height image of (b) pristine NTS (scale bar, 2 μm) and (c) PVA-coated core/shell NTS nanoplatelets on freshly cleaved mica (scale bar, 2 μm), with (d) the corresponding section analysis. Figure 1: Preparation of artificial nacre and AFM characterization of NTS nanoclay before and after coating with PVA. ( a ) Artificial nacre via concentration-induced self-assembly of polymer-coated nanoclay platelets with intrinsic hard/soft architecture. Well-defined core/shell particles are isolated by centrifugation and redispersion. Different aspect ratios are indicated as diameter to thickness ( d / t ) and corresponding fracture modes are displayed to the right as influenced by the aspect ratio and polymer content. ( b , c ) AFM height image of ( b ) pristine NTS (scale bar, 2 μm) and ( c ) PVA-coated core/shell NTS nanoplatelets on freshly cleaved mica (scale bar, 2 μm), with ( d ) the corresponding section analysis. Full size image Table 1 gives an overview of the used nanoclays. Since we focus on the effects of aspect ratio on structure formation and properties, it is of high importance to carefully assess the average size and its distribution. Much of the current understanding of the size distribution of nanoclays relies on scattering and laser diffraction techniques [48] , [49] , [50] . Yet, these techniques only give an indirect measure and are complicated to apply owing to the inherent size distribution, the anisometric/non-circular shape and possible bending of the particles [51] . Commonly used atomic force microscopy (AFM) faces difficulties to provide a statistically valid analysis due to the small scan area [52] , [53] , [54] . Therefore, we invested considerable efforts to realize a statistically relevant real-space analysis of the nanoclay dimensions via scanning and transmission electron microscopy (SEM/TEM) imaging. We refer to the Supplementary Fig. 1 for representative SEM micrographs and to Table 1 for the derived size distributions. In case of the ultrasmall laponite (LAP), being one of the most thoroughly characterized nanoclays, neither TEM nor SEM led to sufficiently robust results and we confirmed the known value from literature [55] with dynamic light scattering ( Supplementary Fig. 2 ). Overall, the synthetic nanoclays display a wide range of aspect ratios from a few tens of nanometres (LAP) via several hundreds of nanometres (SUM, MTM, NHT) up to several micrometres (NTS). We emphasize that NTS even displays sheets in the range of more than tens of micrometres, thus being highly appealing for gas barrier materials, that crucially depend on having ultrahigh aspect ratio nanoplatelets. The imaging data of SUM and NHT reveal some differences with the literature values [56] . We find that SUM is larger and NHT is smaller in size than the reported value. Table 1 Overview of used synthetic nanoclays. Full size table We used AFM to directly visualize the successful coating of PVA in the core/shell nanoplatelets. The height profiles change from ca. 1 nm (pristine nanoclay, see also Supplementary Fig. 5 ) to 2–2.2 nm (PVA-coated nanoclay) in case of the exemplarily depicted NTS, thus confirming the presence of a thin adsorbed polymer layer ( Fig. 1b–d ). AFM also verifies the absence of unwanted aggregation and absence of excess free polymer. We initially compared two preparation methods for the nacre-mimetic films: (i) simple film casting via free water evaporation and (ii) water removal through a filtration membrane, a process similar to paper-making. Both procedures lead to macroscopic and self-standing films, typically prepared with thicknesses of 10–100 μm. Whereas both methods yield films with similar mesostructure for the small nanoclays (LAP and SUM), the films based on the larger nanoclay (NHT and NTS) exhibit a better order of the mesostructure with well aligned flat nanoplatelets after solution casting. Vacuum-filtrated films display a comparably wavy mesostructure ( Supplementary Fig. 3 ). Such microscopic imperfections can lead to grain boundaries, unwanted light scattering and reduced transparency. Therefore, we focus exclusively on solution casting. The self-alignment of large aspect ratio polymer-coated nanoclays can be rationalized due to the formation of nematic liquid-crystalline phases, whose critical concentration depends on the aspect ratio ( Supplementary Fig. 4 ) [56] , [57] . For the ultrasmall PVA-coated LAP nanoclay, the behaviour is however less self-evident, as the cationic rim regions can in principle interact with the anionic basal planes to form edge-on-plane structures, also known as ‘house of cards’ structure [48] , [58] . Therefore, we carefully analysed the mesoscale order using SEM, TEM and 1D/2D X-ray diffraction (XRD). SEM clearly reveals a layered arrangement of the nanoplatelets for all nacre-mimetics starting from PVA/SUM, confirming the successful hydrodynamic self-ordering of the polymer-coated nanoclays during water removal ( Fig. 2 ). In case of ultrasmall LAP platelets, the SEM image shows assemblies of nanoclays protruding from the surface, as individual platelets cannot be identified due to their small size. Below, we will further evidence an in-plane ordering of PVA/LAP films using 2D XRD ( Fig. 3c,d ). For the larger nanoclays individual nanoclay layers are easily visible and the SEM images reflect the increasing platelet size in the following order SUM<NHT<NTS. TEM images of microtomed ultrathin cross sections of selected nanocomposites confirm the presence of alternating hard/soft layers, as quantified by grey scale and Fourier Transform analysis of the samples revealing the characteristic distances. Although the distances may be altered during the microtoming and imaging procedure, the variation between the nanoplatelets serves as an indication for the actual distribution of gallery spacings, which mostly scale between±0.15 nm around the average. 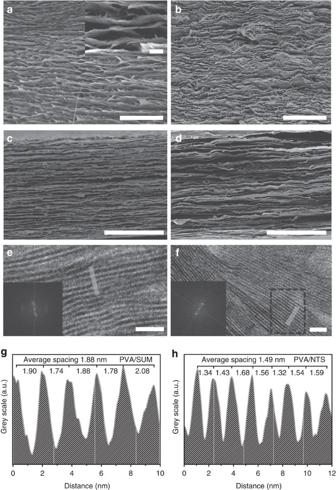Figure 2: Electron microscopy characterization of the cross sections. SEM images of (a) PVA/LAP (scale bar, 2 μm; inset at higher magnification and scale bar, 250 nm), (b) PVA/SUM (scale bar, 2 μm), (c) PVA/NHT (scale bar, 5 μm), (d) PVA/NTS (scale bar, 5 μm) showing a layered ordered arrangement of the nanoclays, embedded in a nanoconfined PVA matrix. SEM images clearly show the increase of platelet size fromatod. TEM images of ultrathin cross sections of (e) PVA/SUM and (f) PVA/NTS (scale bar, 10 nm) showing alternating hard and soft layers. The dark and grey lines correspond to nanoclay and polymer, respectively. Fourier transform analysis of the sample (e) or marked area of the sample (f) are shown as insets. (g,h) Grey scale analysis to quantify the distance between alternating layers. Figure 2: Electron microscopy characterization of the cross sections. SEM images of ( a ) PVA/LAP (scale bar, 2 μm; inset at higher magnification and scale bar, 250 nm), ( b ) PVA/SUM (scale bar, 2 μm), ( c ) PVA/NHT (scale bar, 5 μm), ( d ) PVA/NTS (scale bar, 5 μm) showing a layered ordered arrangement of the nanoclays, embedded in a nanoconfined PVA matrix. SEM images clearly show the increase of platelet size from a to d . TEM images of ultrathin cross sections of ( e ) PVA/SUM and ( f ) PVA/NTS (scale bar, 10 nm) showing alternating hard and soft layers. The dark and grey lines correspond to nanoclay and polymer, respectively. Fourier transform analysis of the sample ( e ) or marked area of the sample ( f ) are shown as insets. ( g , h ) Grey scale analysis to quantify the distance between alternating layers. 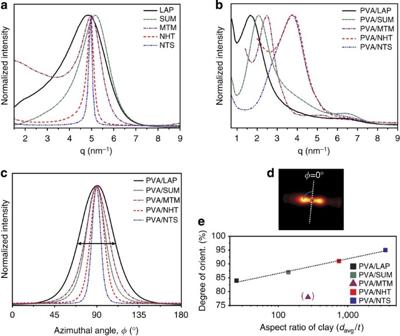Figure 3: XRD characterization of the nanostructure of the layered nacre-mimetics. 1D XRD of (a) pure nanoclays and (b) nacre-mimetic materials. (c) Azimuthal intensity distribution profiles of the primary diffraction peak extracted from 2D XRD. Intensities are normalized to the peak maximum, (d) 2D XRD image of PVA/LAP at 10–15° beam inclination with respect to the plane of the film, (e) The degree of orientation calculated from the full-width at half maximum according to equation (5) for all nacre-mimetics. The value for nacre-mimetics based on natural MTM is shown in brackets, as it is clearly outside of the trend for the materials based on synthetic nanoclays, and neglected for the linear fit. Full size image Figure 3: XRD characterization of the nanostructure of the layered nacre-mimetics. 1D XRD of ( a ) pure nanoclays and ( b ) nacre-mimetic materials. ( c ) Azimuthal intensity distribution profiles of the primary diffraction peak extracted from 2D XRD. Intensities are normalized to the peak maximum, ( d ) 2D XRD image of PVA/LAP at 10–15° beam inclination with respect to the plane of the film, ( e ) The degree of orientation calculated from the full-width at half maximum according to equation (5) for all nacre-mimetics. The value for nacre-mimetics based on natural MTM is shown in brackets, as it is clearly outside of the trend for the materials based on synthetic nanoclays, and neglected for the linear fit. Full size image We used 1D XRD to quantify the interlayer spacing of the layered biomimetic nanocomposites ( Fig. 3a,b ). For better comparison, we first recorded the diffractograms of self-standing films of pristine nanoclays. LAP and SUM show rather broad peaks, indicating comparably small-ordered domains formed by such nanoclays with low aspect ratios. The d *-spacings of LAP and SUM are 1.29 nm [59] and 1.21 nm, respectively. On the contrary, sharp peaks can be obtained for the higher aspect ratio nanoclays, NHT and NTS, with d *-spacings at 1.26 nm for both [56] . MTM with an intermediate aspect ratio displays a broader peak corresponding to its hydrated d *-spacing of 1.26 nm (ref. 45 ). For the nacre-mimetics, we find an unexpected dependence of the primary diffraction peak with the aspect ratio of the nanoclay. The diffractograms ( Fig. 3b , individual comparisons in Supplementary Fig. 6 ) clearly show a shift towards higher scattering vector q with an increasing aspect ratio. The corresponding d *-spacings can be calculated to range between 3.7 to 1.7 nm when passing from the smallest LAP to the largest NTS. Weak and broad humps appear as integer multiples of the primary peak ( n ·q *) corresponding to the higher-order peaks characteristic of a lamellar morphology. The XRD shows no peak for non-exfoliated synthetic nanoclays in the nanocomposites, thereby indicating a near quantitative activation of the nanoclay surface during the coating procedure. However in case of PVA/MTM, a small broad hump appears at q ~5.3 nm −1 indicating small traces of non-exfoliated MTM in the nanocomposite rooted from the difficulty of the exfoliation of natural clays and demonstrating the need for proper fractionation. Additional 2D XRD of PVA/LAP eliminates any ambiguity on the alignment of its mesostructure by demonstrating strongly confined diffraction arcs originating from a highly ordered structure, regardless of the small aspect ratio ( Fig. 3d ). The degree of orientation ( Π ) can be calculated from the full-width half maximum according to equation (5) to be as high as 84% (see methods). The same analysis of the 2D XRD data for PVA/NTS containing nanoplatelets with a three order of magnitude larger aspect ratio reveals increased alignment with a very high degree of orientation close to 95%. In fact the degree of orientation follows a close to linear dependence in the semi-logarithmic plot when considering all synthetic nanoclays ( Fig. 3e , Table 2 ). On the contrary, nacre-mimetics based on natural MTM show a lower degree of alignment, likely owing to inhomogeneities hampering a perfect structure formation. The trend can be related to the increased propensity of larger aspect ratio nanoclays to form ordered nematic, liquid crystalline phases and demonstrates a clear advantage for the structure-formation process. Overall, it is important to realize that the values for all samples based on synthetic nanoclays scale within 10% and thus they are similarly aligned to a very high degree. Table 2 Structural characterization of various nacre-mimetics. Full size table To further understand the observed differences in lamellar periodicities of the nacre-mimetics, we determined their elemental composition by elemental analysis. Here, a similar trend is observed, yielding the highest polymer content for the smallest nanoclay ( ca. 58 wt% in PVA/LAP), while the highest aspect ratio nanoclays only contain less than half of this ( ca. 24 wt% in PVA/NTS). PVA/MTM displays an intermediate polymer content of ca. 38 wt%. This trend is also fully reflected in thermogravimetric analysis, where degradation above 300 °C is observed ( Table 2 , Fig. 4c ). 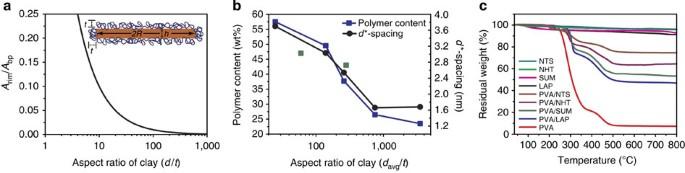Figure 4: Polymer content andd*-spacing of the nacre-mimetics as a function of the nanoclay aspect ratio. (a) Change in ratio of surface area of rim to basal planes with increasing size of the nanoclay platelets. The amount of polymer adsorbed at the rim becomes insignificant for increasingly larger nanoclays. (b) Dependence of polymer content andd*-spacing on the aspect ratio of all the nanoclays including fragmented NTS with smaller aspect ratios of 280 and 60 (dark cyan symbols). (c) Thermogravimetric analysis of pristine nanoclays and the corresponding nacre-mimetic hybrid films. Figure 4: Polymer content and d *-spacing of the nacre-mimetics as a function of the nanoclay aspect ratio. ( a ) Change in ratio of surface area of rim to basal planes with increasing size of the nanoclay platelets. The amount of polymer adsorbed at the rim becomes insignificant for increasingly larger nanoclays. ( b ) Dependence of polymer content and d *-spacing on the aspect ratio of all the nanoclays including fragmented NTS with smaller aspect ratios of 280 and 60 (dark cyan symbols). ( c ) Thermogravimetric analysis of pristine nanoclays and the corresponding nacre-mimetic hybrid films. Full size image In principal these differences can either be attributed to different polymer/clay interactions (slightly different surface energies for the various nanoclays), or to geometrical reasons because higher rim-to-surface ratios for lower aspect ratio nanoclays lead to larger fractions of adsorbed polymer. Let us first rationalize the geometrical constraints using a simple model for disc-shaped nanoclays, taking into account the radius and height of the nanoclay, R and h , and the polymer volume, V bp and V rim , adsorbed at the two basal planes and around the rim, with the surface areas, A bp and A rim . A constant thickness, t , is assumed for the polymer coating. Equation (1) describes the ratio of polymer volume adsorbed at the rim versus adsorbed on the two basal planes. This ratio scales with R −1 , meaning that the polymer volume adsorbed at the rims becomes progressively smaller at constant total surface area of the basal planes for increasing radius of the considered individual platelets ( Fig. 4a ). The total polymer volume ( V pc ) on a single nanoclay platelet is the sum of the volume adsorbed at both basal planes and the rim and can be expressed as, By combining the equations, we can express the ratio of polymer volume at rim to the total volume of polymer coating as follows, Equation (4) similarly shows that smaller nanoplatelets have higher volume of polymer adsorbed at the rims. This ratio even enlarges when coverage at the rim area is favored over adsorption at the basal planes. Such a phenomenon is in fact reported for LAP, the best characterized synthetic clay, for which small-angle neutron scattering demonstrated a higher thickness of the polymer coating at the rim areas versus the basal planes [55] . Figure 4a illustrates how the ratio of the surface area of the rim versus that of the basal plane decreases with increasing radius (nanoclay size). Interestingly, these scaling dependences are independent of the actually adsorbed thickness of the polymer layer, t . Since the height of the used nanoclay platelets is nearly constant ( h ~1 nm), the scaling dependence is valid for different nanoclays. Certainly, different surface energies owing to the different chemical compositions of the nanoclays may also play a role in the adsorptive layer. To investigate this effect, we used a high-shear microfluidizer to fragment the large NTS nanoclay and prepared nacre-mimetics from two smaller-sized NTS batches (PVA/NTS 280 and PVA/NTS 60 ; subscript indicates aspect ratio by SEM). Indeed we also find increasing polymer content for smaller nanoclay batches with the same surface energy as the parent nanoclay (NTS 3500 ). Hence, the geometrical model mostly explains the higher polymer content in PVA/LAP and PVA/SUM compared with the nacre-mimetics with larger nanoclays. Interestingly, for these differences in polymer content to translate into larger gallery spacings, the polymer content needs to be at least partly pushed into the gallery spacings during self-assembly process, possibly due to lateral contraction in the late stages of water evaporation. This becomes increasingly difficult for larger nanoclays, which can be seen in the near constant d *-spacing for the higher aspect ratio nanoclays (NHT and NTS). Fig. 4b compares the d *-spacing from XRD with the polymer content from elemental analysis and establishes a correlation between both characteristics. Mechanical properties Next, we will discuss the mechanical properties as a function of aspect ratio, and viscoelastic properties of the polymer layer and its thickness ( Figs 5 , 6 and Supplementary Table 1 ). Previous experiments on clay-based nacre-mimetics almost exclusively focused on MTM as building block and hardly any data for mechanical properties is available for other aspect ratios or synthetic nanoclays [27] , [28] , [38] , [60] , [61] . Establishing these relationships and understanding the fracture mechanisms for biomimetic materials, in particular involving polymers under nanoconfinement, are however vital to provide the foundation for future rational design and the ability to target performance maxima. Here, we focus mainly on a comparison of the properties of nacre-mimetics based on synthetic nanoclays and only relate at selected parts to previously investigated PVA/MTM materials. The influence of aspect ratio is intuitively anticipated owing to the fact that yielding of a composite material can more easily occur for lower aspect ratio nanoclays and higher fractions of polymer, while stiffness is favored for larger aspect ratio nanoclays and highest fraction of reinforcements. These relationships were successfully established for fibre-reinforced composites and classical nanocomposites, but have not been shown to be applicable for highly reinforced nacre-mimetics that are controlled to a large extent by interfaces and involve the nanoconfinement of the polymer layers. For simplicity, we have to make the reasonable assumption that the intrinsic stiffness of the various nanoclays and the interfacial stress transfer of the polymer onto the nanoclays are on a similar level. We believe this to be fair as we are dealing with the same material class with only small changes in the composition. To further support this assumption, we also later on discuss nacre-mimetics based on fragmented clay samples, thereby using exactly the same nanoclay but with different aspect ratios (PVA/NTS with d / t =3,500, 280, 60). We also discuss humidity-dependent studies to add crucial complementary information on the influence of the dynamics of the nanoconfined polymer on the macroscale mechanical properties. We refer to the Supplementary Table 1 for the list of all data on mechanical properties. 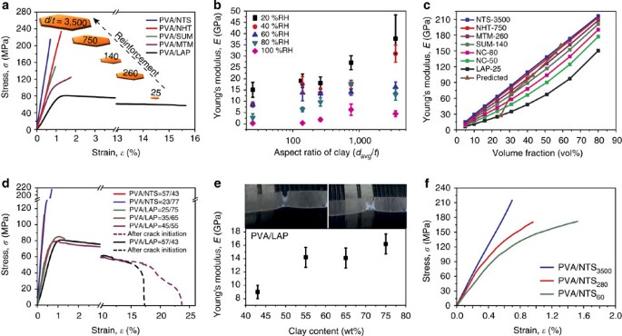Figure 5: Tensile mechanical properties of nacre-mimetics. (a) Influence of the aspect ratio of nanoclays on tensile mechanical properties measured at 40 %RH for nacre-mimetics prepared from isolated core/shell particles. (b) Dependence of Young’s modulus of nacre-mimetics on the aspect ratio of nanoclay at different %RH (see alsoFig. 6). (c) Variations of Young’s modulus with volume fraction of reinforcement are shown for different aspect ratios following the Halpin−Tsai model, consideringEm=2.3 GPa at 40 %RH (see alsoSupplementary Note 1),Er=270 GPa andt=1 nm (NC=nanoclay). The predicted values for our nacre-mimetics are added, considering the actual polymer content and the aspect ratio of the individual nanoclay. (d) Influence of polymer content on tensile mechanical properties for PVA/NTS and PVA/LAP (40 %RH, polymer content indicated in w/w within the panel). Dotted lines indicate stable crack propagation. (e) Dependence of Young’s modulus of PVA/LAP on polymer content. Photographs of PVA/LAP=45/55 sample show the crack initiation and stable crack propagation. (f) Effect of platelet size of fluidized/fragmented NTS nanoclay on tensile mechanical properties of corresponding nacre-mimetics based on perfect core/shell particles. Figure 5: Tensile mechanical properties of nacre-mimetics. ( a ) Influence of the aspect ratio of nanoclays on tensile mechanical properties measured at 40 %RH for nacre-mimetics prepared from isolated core/shell particles. ( b ) Dependence of Young’s modulus of nacre-mimetics on the aspect ratio of nanoclay at different %RH (see also Fig. 6) . ( c ) Variations of Young’s modulus with volume fraction of reinforcement are shown for different aspect ratios following the Halpin−Tsai model, considering E m =2.3 GPa at 40 %RH (see also Supplementary Note 1 ), E r =270 GPa and t =1 nm (NC=nanoclay). The predicted values for our nacre-mimetics are added, considering the actual polymer content and the aspect ratio of the individual nanoclay. ( d ) Influence of polymer content on tensile mechanical properties for PVA/NTS and PVA/LAP (40 %RH, polymer content indicated in w/w within the panel). Dotted lines indicate stable crack propagation. ( e ) Dependence of Young’s modulus of PVA/LAP on polymer content. Photographs of PVA/LAP=45/55 sample show the crack initiation and stable crack propagation. ( f ) Effect of platelet size of fluidized/fragmented NTS nanoclay on tensile mechanical properties of corresponding nacre-mimetics based on perfect core/shell particles. 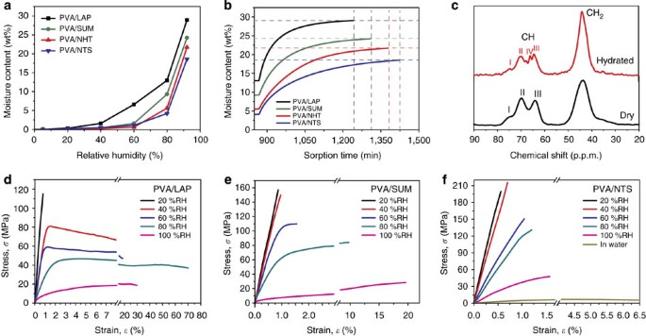Figure 6: Influence of humidity on nacre-mimetics based on core/shell particles. (a) Moisture content of nacre-mimetics as a function of relative humidity at 28 °C. (b) Kinetics of moisture sorption from 80 to 92 %RH. (c)13C-CPMAS NMR spectroscopy study of PVA/LAP at 23 °C in dry state and in hydrated state by soaking in D2O. A characteristic rubbery peak (IV) at 66 p.p.m. is obtained for hydrated PVA/LAP, while it remains absent in the dry materials. (d–f) Influence of humidity on tensile mechanical properties of PVA/LAP, PVA/SUM and PVA/NTS, respectively. Full size image Figure 6: Influence of humidity on nacre-mimetics based on core/shell particles. ( a ) Moisture content of nacre-mimetics as a function of relative humidity at 28 °C. ( b ) Kinetics of moisture sorption from 80 to 92 %RH. ( c ) 13 C-CPMAS NMR spectroscopy study of PVA/LAP at 23 °C in dry state and in hydrated state by soaking in D 2 O. A characteristic rubbery peak (IV) at 66 p.p.m. is obtained for hydrated PVA/LAP, while it remains absent in the dry materials. ( d – f ) Influence of humidity on tensile mechanical properties of PVA/LAP, PVA/SUM and PVA/NTS, respectively. Full size image Focusing first mainly on the elastic properties ( Fig. 5a,b ), it is seen that nacre-mimetics based on the largest synthetic nanoclays (PVA/NTS) show drastically higher stiffness with a Young’s modulus close to 40 GPa at 20 %RH, which is approaching that of natural nacre (E=40–60 GPa in wet and 70 GPa in dry conditions [3] , [4] ). At the same time this material reaches a tensile strength of 200 MPa, which is double or triple of that of natural nacre. Most importantly, the ultrahigh aspect ratio of NTS allows reaching stiffness values significantly higher than what can be achieved with natural MTM. PVA/NTS in fact realizes values that have previously only been achievable using covalent [36] , [62] or supramolecular crosslinking [15] , [40] . Hence, there is a clear and profound advantage of exploiting larger aspect ratio nanoclays, giving a fresh impulse for the proper selection in future nacre-mimetics. In general, a loss in stiffness is observed for decreasing the aspect ratio. This loss in stiffness can however not only be associated with the lower aspect ratio of the nanoclay, but also needs to take into account the lower weight fractions of inorganic reinforcements as found in elemental analysis, thermogravimetric analysis and XRD ( Fig. 4 ). To allow a better understanding, we calculated the Young’s moduli for selected aspect ratios and as a function of the reinforcement content (vol%, Fig. 5c ). These calculations are on the basis of Halpin−Tsai [63] , [64] model developed for layered nanocomposites oriented in tension direction [65] . We refer to the SI for the Jaeger−Fratzl model and the modified Halpin−Tsai model comparing systems with parallel and random orientation, respectively ( Supplementary Fig. 7 and Supplementary Note 1 ) [64] . From this plot, we see that (i) increasing the volume fraction of nanoclay induces higher stiffness and (ii) larger aspect ratio nanoclays lead to higher stiffness at the same level of reinforcement. However, it also becomes evident that there is no further significant improvement in Young’s modulus upon increasing the aspect ratio once a critical aspect ratio is reached at a particular volume fraction of nanoclay (vertical dependence). This is simply because stress transfer already fully activates the nanoplatelets after a critical size. In our nanocomposites, we find higher reinforcement contents when increasing the nanoclay aspect ratio. Therefore, the higher stiffness obtained for nacre-mimetics with larger nanoclays is not only because of increasing aspect ratio of the reinforcement but also because of containing higher fractions of it (see predicted values). In addition, larger synthetic clays benefit from a slightly better in-plane orientation ( Fig. 3e , Table 2 ). This can however only be considered as a minor contribution to enhancing unidirectional stiffness as the degree of orientation for all synthetic nacre-mimetics scale within 10%, whereas the aspect ratios change by three orders of magnitude. The experimental stiffness values are lower than predicted by the Halpin−Tsai and Jaeger−Fratzl models ( Fig. 5c , and Supplementary Fig. 7 ). This is yet a common phenomenon in nanocomposites and originates from the inefficient stress transfer, from the matrix to the nanoclay, not allowing to realize the full potential of the nanoclay reinforcement. A discontinuity is observed when comparing PVA/MTM and PVA/SUM ( Fig. 5a ). Although natural MTM has a slightly higher aspect ratio, the resulting nacre-mimetic displays lower stiffness than PVA/SUM and also an onset of yielding. This is particularly interesting, considering that PVA/SUM contains almost 12 wt% more PVA. We associate the higher stiffness to the advantages of synthetic nanoclays, which display better exfoliation and a better adsorption of polymers owing to a more homogeneous surface chemistry, therefore allowing better stress transfer and higher cohesive strength. In addition the degree of orientation is substantially lower for the PVA/MTM film, leading to a less efficient unidirectional reinforcement (see Fig. 3e ). The lower stiffness of solution cast PVA/MTM in this paper as compared with previous PVA/MTM films prepared by vacuum filtration [42] is attributed to the presence of 8 wt% more polymer in the cast film, different nanoclay fractionation and batch (natural product), and unlike structure-formation processes associated with the different preparation methods. While vacuum filtration leads to a forced concentration increase at the surface of the filtration unit and an asymmetric structure development, free film casting mostly leads to a homogeneous increase of the concentration of the core/shell platelets. Upon passing a critical concentration, a liquid-crystalline state develops, which then becomes arrested during final drying. Different lateral stress occurs during final stages of drying. Concerning the tensile strength, a similar trend can be observed in the nacre-mimetics. Although tensile strength is governed by defects in case of linear elastic materials, we observe an increase in tensile strength as the size of the nanoclay (and concurrently the fraction of reinforcements, Table 2 ) enlarges, and reach a maximum of 200 MPa at 20 %RH for superlarge NTS nanoclay. We relate the observation of this consistent trend to similar amounts of detrimental defects owing to analogous preparation conditions for all nacre-mimetics. A direct comparison of all nacre-mimetics at 40 %RH ( Fig. 5a ) reveals a prominent transition in terms of the deformation modes when passing from highest to lowest aspect ratio nanoclays. We chose 40 %RH for this comparison, as the water uptake due to the humidity is similar for all nacre-mimetics at this point ( Fig. 6a ). Interestingly, PVA/LAP shows a clear and pronounced onset of yielding. This preferential yielding is caused by the comparatively higher fraction of polymer, and more importantly, by the lower aspect ratio of the nanoclay allowing a transition of the deformation mode from platelet fracture to platelet pull-out, as also seen in SEM ( Fig. 2a ). A more global understanding of the mechanical behaviour depending on the size and type of synthetic nanoclay should also include (i) the influence of the polymer content on the yielding and mechanical properties for differently sized nanoclays and (ii) analysing the effect of potentially different adsorption strength of polymers on nanoclays of different chemical composition. We address the first objective by varying the polymer fraction in nacre-mimetics based on smallest (LAP) and largest (NTS) nanoclays from the values found in their corresponding materials based on ‘perfect’ core/shell particles (PVA/LAP=58 wt% PVA; PVA/NTS=24 wt% PVA). This can be achieved by careful direct mixing [44] and subsequent film casting. Let us first focus on PVA/LAP prepared at different polymer fractions. Structural characterization by XRD shows lower gallery spacing for less polymer, hence confirming a smooth and adequately defect-free structure build-up also at lower fractions of polymer ( Supplementary Fig. 8 ). The corresponding tensile-testing curves for PVA/LAP show a similar yielding transition down to a polymer content of 35 wt% ( Fig. 5d ). For comparison, PVA/SUM ( d / t =140, 50 wt% polymer content) does not show inelastic deformation under similar conditions, hence demonstrating a first clear influence of the nanoclay size on the transition to inelastic deformation. Upon further reduction of the polymer content down to the level of PVA/NTS (25 wt%), the inelastic deformation is lost. This demonstrates that a minimum layer thickness of the nanoconfined polymer is necessary to allow inelastic deformation ( d *>2.4 nm, Supplementary Fig. 8 ) for small LAP. To correlate this behaviour from the other end, we also prepared PVA/NTS with a higher polymer content similar to PVA/LAP (labelled as PVA/NTS=57/43). The corresponding tensile-testing curve however, still shows purely linear elastic behaviour, and also some lower tensile strength, possibly due to a different level of defects. In summary, all of these comparisons demonstrate that the size of the nanoclay is crucial in deciding over the presence of inelastic deformation (at the same polymer content) and that toughness is favored for smaller nanoclays. Interestingly enough we find stable crack propagation through the PVA/LAP materials down to a polymer content of ca. 45 wt%, and one can observe a large process zone (stress whitening) around the propagating crack tip, even at only 40 %RH ( Fig. 5e ). This shows efficient distribution of fracture energy and is a clear indication of enhanced toughness. The polymer content of 45 wt% can be considered as optimum for PVA/LAP as the higher amount of reinforcement also increases the stiffness to 14 GPa, without sacrificing inelastic deformation. We study the second objective—effect of interfacial adsorption energy—for different sizes of the same nanoclay after fragmentation using a microfluidizer. We focus on two batches with aspect ratios of 280 and 60, complementing the existing PVA/NTS 3,500 material with aspect ratio 3,500. The tensile curves of the corresponding nacre-mimetics show the same decrease of the elastic properties and an onset of yielding for the material containing the smallest batch of NTS (PVA/NTS 60 ) ( Fig. 5f ). This behaviour is very similar to what has been found earlier when varying the nanoclay aspect ratio by changing the type of nanoclay ( Fig. 5a ), and corroborates the relationships discussed above. To better understand the deformation mechanisms as a function of the viscoelastic properties of the polymer, we further studied the effect of humidity on the mechanical properties of the nanocomposites based on the pure core/shell particles ( Fig. 6 ). Fig. 6a quantifies the water uptake by water sorption experiments for the various nacre-mimetics. One observes a similar and rather low water uptake for all nacre-mimetics till around 40 %RH. Upon further increase of the relative humidity, the sorption curves start to deviate and the nacre-mimetics with smaller nanoclays contain more water because of the higher polymer content. The overall differences range however in a narrow window of only 10%. The kinetics of water uptake for the increase from 80–92 %RH reveal a faster mass increase and an earlier equilibration for smaller nanoclays ( Fig. 6b ). This reflects the barrier properties of the materials, because water molecules have a larger tortuous pathway and hence slower migration perpendicular to the materials for largest aspect ratio nanoclays, while the diffusion of water molecules is comparably quick for smaller nanoclays. In terms of mechanical properties, a softening in the elastic region is common to all materials due to the plasticizing effect of water ( Fig. 6d–f ; Fig. 5b ). In strong contrast are however the differences in inelastic deformation. The tensile curves at different %RH clearly show that PVA/LAP and PVA/NTS serve as the two extremes, while PVA/SUM takes the intermediate position in demonstrating the switch over in behaviour from elastic to plastic deformation with increasing humidity ( Fig. 6d–f , Supplementary Table 1 ). This trend clearly originates from the aspect ratio of the used nanoclay. While humidity significantly increases the ductility of the materials with lower aspect ratio nanoclay (LAP and SUM) and leads to an increase of the elongation at break ( ε b ) from below 1% (20 %RH) to 30% (100 %RH), inelastic deformation is almost absent for the largest aspect ratio nanoclays (NHT and NTS) up to 100 %RH. The pronounced yielding and inelastic deformation for PVA/LAP and PVA/SUM takes place by frictional sliding of small nanoclay platelets owing to softening and lower internal cohesion of the polymer with increasing levels of internal hydration. This can be traced by solid-state 13 C cross-polarization magic-angle spinning nuclear magnetic resonance ( 13 C-CPMAS NMR) for the nacre-mimetic with the highest polymer content (PVA/LAP) and for the two extreme cases of hydration, that is, dehydrated and hydrated ( Fig. 6c ). The hydrated sample clearly shows the appearance of an additional peak at 66 p.p.m. in the region of the α-carbon (-CH 2 - C HOH-; labelled as (IV)). This peak is associated with a rubbery character and enhanced chain dynamics of PVA, as opposed to pure glassy character found at low relative humidity [66] . PVA/LAP yields earlier and more than PVA/SUM owing to (i) the lower aspect ratio of the LAP nanoclay leading to less efficient reinforcement and easier platelet pull-out and (ii) its higher polymer content compared with PVA/SUM enhancing dynamics and interfacial slippage. Further differences can be seen in the slopes of the tensile-testing curves in the plastic region. Contrary to PVA/SUM, PVA/LAP shows a drop in strength after the yield point for most humidities. This decrease derives from slight necking, which can exclusively be observed for PVA/LAP. Larger nanoclays in their corresponding nacre-mimetics (PVA/NHT and PVA/NTS) provide higher reinforcement and stiffness, leading to almost purely elastic deformation. This is because of the presence of minimal amounts of polymer, which is completely nanoconfined between stacked ultralarge nanoclays ( d *~1.7 nm). Significant inelastic deformation can only be observed upon full plasticization when placed into water. Correspondingly, the modulus of toughness or work-of-fracture, as measured by the area under the curves strongly depends on the deformation mechanisms and tendency for inelastic deformation. While the largest aspect ratio nanoclays show only minimum increase in work-of-fracture, the PVA/LAP and PVA/SUM materials show drastically enhanced toughness enabled by yielding at 40 and 80 %RH, respectively. As mentioned above, PVA/LAP also shows stable crack propagation. With respect to other known nacre-mimetics [11] , [32] , [37] , [39] , [60] , [61] , [67] , PVA/LAP based on pure core/shell platelets and its optimized variant with slightly less polymer (PVA/LAP=45/55, see Fig. 5d ) demonstrate good stiffness close to 10 and 15 GPa, good tensile strength and at the same time realize a substantial work-of-fracture of 10±3.2 MJ m −3 and 15±6.5 MJ m −3 at 40 %RH, respectively. Owing to the more pronounced inelastic deformation this value increases up to 31±7.5 MJ m −3 at 80 %RH, albeit compromising stiffness and strength. A similar trend and values are found for PVA/SUM, but with a transition at higher %RH, implying that depending on the application conditions the appropriate nanoclay needs to be selected. Transparency and gas barrier as functional properties In terms of developing multifunctional property profiles for functional biomimetic materials, synthetic nanoclays represent viable advantages, especially when aiming at fully transparent and highly flexible coatings and self-standing films with outstanding barrier properties. Such materials are intensely needed as flexible encapsulants or substrates for (printable) organic electronics, or for gas storage applications. The primary factors promoting gas barrier are increasing the nanoclay aspect ratio, as well as the nanoclay fraction, exfoliation and orientation in the nanocomposite, and diminishing free volume. Nacre-mimetics fulfil most criteria to the best possible extent, yet free volume remains difficult to predict and to experimentally access. For full transparency, grain boundaries and irregularities in the self-assemblies must be prevented to reduce detrimental light scattering within the film. At the same time, the surface must be of high quality containing minimum roughness to avoid surface scattering. First, let us focus on the transparency of our materials. The optical properties of the films are remarkable in terms of transparency, when properly treated (see below). Again, a clear size effect can be deduced, separating the smaller aspect ratio nanoclays from the ones with high aspect ratio. The photograph of PVA/LAP depicts a film with basically full, glass-like transparency and high optical clarity ( Fig. 7a ). PVA/LAP films transmit 95–97% of the spectrum of the visible light at a film thickness of ca. 25 μm and PVA/SUM films show 85–92% transmittance for the same film thickness. The best similar materials prepared from natural MTM and PVA only show a transmittance of 33–67% at normalized thickness of 25 μm [36] . On the contrary, some unexpected difficulties are encountered for the nacre-mimetics with higher aspect ratio nanoclays, NHT and NTS. Both materials do not reach the optical clarity of PVA/LAP and PVA/SUM, and typically only show translucent films. Careful SEM investigations reveal at least one origin by visualizing a ca. 1.5–2 μm thick heterogeneous skin layer, which forms during evaporation of the dispersion (see Fig. 7e , Supplementary Fig. 9 ). This layer causes surface scattering and leads to a certain opaqueness, while the interior and bottom of the film are perfectly structured as seen by SEM. To overcome the detrimental surface scattering, we applied a very thin clear coat ( ca. 3 μm, Supplementary Fig. 10 ) matching closely the refractive index of the nacre-mimetic to reduce interfacial scattering by providing a smooth top surface ( Fig. 7c–f ). This leads to a substantial increase of the transmittance as seen in the photographs and transmission measurement. Yet the transparency after applying the clear coat cannot reach the near perfect optical quality of the films prepared from the lower aspect ratio nanoclays (PVA/LAP and PVA/SUM). This points to the need of even further refining the structure formation process, in particular diminishing the presence of the heterogeneous surface layer using highly tailored polymers and also understanding the contribution of scattering by individual superlarge nanoplatelets within the film. Overall, the synthetic nanoclays provide a substantial improvement, pushing the application areas of mechanically superior and thick nacre-mimetic films into fields where highest transparency is desirable. 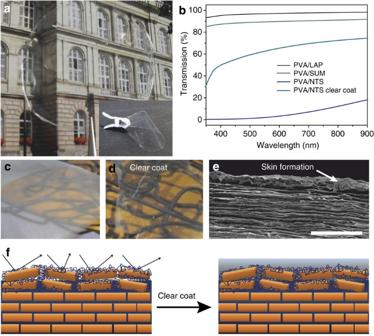Figure 7: Optical properties of nacre-mimetics based on synthetic nanoclays with various aspect ratios. (a) Photographs of an almost fully transparent PVA/LAP film. (b) Transparency by UV-Visible spectroscopy (normalized to 25 μm thickness). (c,d) Nacre-mimetics with larger nanoclay (PVA/NTS) show translucency, but require a clear-coat matching the refractive index of the nacre-mimetics closely to become almost transparent. (e) SEM depicting the skin formed during preparation of a PVA/NTS nacre-mimetic (scale bar, 5 μm). (f) Schematic (not in scale) showing how a clear coat of matching refractive index diminishes surface scattering by providing a smooth top surface layer. Figure 7: Optical properties of nacre-mimetics based on synthetic nanoclays with various aspect ratios. ( a ) Photographs of an almost fully transparent PVA/LAP film. ( b ) Transparency by UV-Visible spectroscopy (normalized to 25 μm thickness). ( c , d ) Nacre-mimetics with larger nanoclay (PVA/NTS) show translucency, but require a clear-coat matching the refractive index of the nacre-mimetics closely to become almost transparent. ( e ) SEM depicting the skin formed during preparation of a PVA/NTS nacre-mimetic (scale bar, 5 μm). ( f ) Schematic (not in scale) showing how a clear coat of matching refractive index diminishes surface scattering by providing a smooth top surface layer. Full size image We also studied the oxygen permeability being of pivotal importance for applications in barrier materials. Synthetic NTS nanoclay is among the nanoclays with the best ever reported aspect ratio, hence motivating above all to pursue gas barrier properties. In recent years, Ebina and Mizukami [27] obtained a remarkably low oxygen permeability of 0.00074, cm 3 · mm · m −2 · day −1 · atm −1 at dry conditions for a self-standing polymer/clay film. The film was prepared by coordination of 20 wt% poly(sodium acrylate) to the lateral rims of SUM as binder. Although being outstanding in terms of oxygen barrier properties, the films demonstrate poor mechanical properties exhibiting tensile strength of only around 25 MPa [27] , [28] . In addition, sequential LbL of different nanoclays and polymers as ultrathin surface coatings revealed an extraordinary performance, and large hopes arise from new synthetic clays with highest aspect ratios [31] , [54] . However, the LbL method ultimately faces clear limitations when aiming at higher coating thicknesses or even self-standing films. Main advantages of our films are the very good mechanical properties, simple and fast preparation of thick films, and the possibility to measure them directly as freestanding films, hence also eliminating any influence from supporting layers. Table 3 compares all materials at high relative humidity. High relative humidity poses challenging conditions for gas barriers based upon water-soluble polymers, as increased free volume and plasticization allow faster diffusion of gas molecules [32] , [33] , [34] , [37] , [68] . Interestingly, the smaller synthetic nanoclays actually outperform previously investigated PVA/MTM [36] , despite the fact that the weight fraction of nanoclay is lower. In particular PVA/SUM containing the larger nanoclays compared with PVA/LAP shows a one order of magnitude better performance and reaches very low oxygen permeability of 0.056 cm 3 · mm · m −2 · day −1 · atm −1 . A clear further increase of the gas barrier is possible by changing to PVA/NTS containing the largest synthetic clays, that allows to reach superbly low gas permeability of only 0.005 cm 3 · mm · m −2 · day −1 · atm −1 (triple-checked for different films). Such permeability values are better than the commercially available barrier films based on synthetic polymers such as polyvinyl chloride, polyvinyl alcohol, polyethylene terephthalate [69] and even highly oriented ethyl vinyl alcohol at similar humidity [70] . In fact the gas barrier is amongst the best ever reported values for layered clay materials—found here in a self-standing material at 80 %RH [27] , [31] , [32] , [34] , [37] , [54] . Therefore, the unique combination of transparency, gas barrier, and mechanical robustness make these rapidly prepared self-standing nanocomposite films a choice for food packaging, gas storage applications, and as sealants and advanced substrates for flexible organic electronics. The herein demonstrated high gas barrier and glass-like transparency complement our previously shown outstanding fire and heat barrier properties for self-assembled nacre-mimetics [44] . Table 3 Oxygen barrier properties of PVA/nanoclay nacre-mimetics. Full size table We herein established the correlation among structure formation, nanostructuration, mechanical deformation modes and functional properties for self-assembled artificial nacre using synthetic clays bridging three orders of magnitude in aspect ratio. We find that the mechanical properties can be crucially influenced by the size of the nanoclay, ranging from ultrastiff materials for the highest aspect ratio to extremely tough materials with pronounced inelastic deformation for the smallest. These differences are not only because of the different aspect ratios and changes in the failure mode from platelet fracture to platelet pull-out, but also relate to the fact that higher amounts of polymer are present for smaller nanoclay owing to larger fractions of adsorbed polymers in the rim areas. Changing the viscoelastic properties via hydration-induced plasticization enables a further understanding of the changes in fracture behaviour from linear elastic to plastic as a function of humidity and accelerated dynamics, following closely the nanoplatelet size. True advantages of the synthetic nanoclay manifest in practically fully transparent, glass-like nacre-mimetics for the smaller aspect ratio nanoclays, while at the same time showing among the best gas barrier properties known for nacre-mimetics. Together with the advanced mechanical properties, a wide-ranging and advanced multifunctional property profile can be realized. The lower transparency for larger clays is in part because of the formation of a skin layer, which can be diminished using a suitable clear coat. Further improvements in this direction require to clearly characterize the free volume in these materials as a function of the aspect ratio, and that even better suited polymer systems need to be identified to reduce the remaining structural defects and the propensity for skin formation in nacre-mimetics based on the largest aspect ratio nanoclays. This study establishes the needed foundation for future rational design of nacre-mimetics to tune material properties and target highest performance. The combination of advanced and tunable mechanical properties with excellently developed functionalities, allowed by feasible large-scale processing, extends the application prospects of nacre-mimetic materials beyond mechanical properties or the focus on singular functionalities. Advanced multifunctional biomimetics are now in reach, such as high performance, mechanically robust, transparent barrier coatings and self-standing substrates for organic electronics. Materials PVA (M w =85–126 kDa, 98% hydrolyzed; Aldrich); Laponite RD (LAP) and Na-cloisite (MTM, both Rockwood Industries). SUM (Kunimine Industries Co. Ltd.), sodium fluorohectorite (NHT) and sodium tetrasilicic mica (NTS, both Topy Industries Ltd.) were used as received. MilliQ water was used in all experiments. Exfoliation of LAP and SUM and MTM nanoclays LAP and SUM were dispersed in MilliQ water (0.5 wt%) and stirred for 2–3 h to yield completely exfoliated dispersions. MTM was stirred vigorously overnight, then left for 4–5 days to allow sedimentation of large agglomerates, and finally decanted. The homogenous supernatant dispersion was used to prepare the nanocomposites. Exfoliation of NHT and NTS nanoclays Cleaning was done similarly as reported [52] with slight changes in the centrifugation speed and time. A 5 wt% aqueous solution of each nanoclay was centrifuged at 12,000 r.p.m. speed for 90 min. After the centrifugation, the dispersion exhibits three different phases (see Supplementary Fig. 11 ). The middle viscose phase contains the desired clean nanoclay with 10–13 wt% solid content, which was then used to prepare 0.5 wt% exfoliated dispersions. Fragmentation of NTS nanoclays A 5 wt% cleaned NTS dispersion was passed through a microfluidizer (Microfluidicscorp MRT CR5) applying 1,400 bar shear cycles for 10 and 20 passes to obtain two batches of NTS nanoclay dispersion having two different sizes. SEM characterization yields the corresponding aspect ratios to 280 and 60. Preparation of self-standing films of pristine nanoclays A 0.5 wt% exfoliated nanoclay dispersion was poured into petri dishes and dried at ambient conditions. Preparation of nacre-mimetic films via solution casting A 0.5 wt% exfoliated nanoclay dispersion was slowly added to 1 wt% aqueous solution of PVA under continuous magnetic stirring. This process was easily scaled up to 2–4 l and the dispersion was stirred for at least overnight for complete polymer adsorption on the nanoclay surface. Excess polymer was removed by centrifugation at 11,000 r.p.m. (for LAP and SUM) and at 5,000 r.p.m. (for MTM, NHT and NTS), followed by washing (2x) and redispersion in MilliQ water. The dispersions were then poured into petri dishes and dried at ambient conditions. Preparation of nacre-mimetic films by direct mixing and film casting To tailor the weight fractions of PVA/LAP and PVA/NTS to exactly the same values, a 0.5 wt% exfoliated nanoclay dispersion was added slowly to 0.5 wt% aqueous solution of PVA under continuous magnetic stirring until the desired weight ratio was obtained. The dispersion was stirred overnight for complete polymer adsorption on the nanoclay surface, poured into petri dishes and dried at ambient conditions. Field-emission scanning electron microscopy Field-emission scanning electron microscopy was performed on a (i) Hitachi S-4800 field-emission microscope (1.5 kV) after sputter-coating a thin Au/Pd layer on the cross-section of the film and (ii) on a Hitachi SU-9000 (30 kV) both in transmission and scanning mode without sputtering. Thermogravimetric analysis Thermogravimetric analysis was done using a NETZSCH TG 209C instrument under continuous flow of 25 ml min −1 of N 2 at a heating rate of 20 K min −1 . Atomic force microscopy Atomic force microscopy was performed on a Veeco Multimode in tapping mode conditions using standard silicon cantilevers (PPP-SEIH-W from Nanosensors). Transmission electron microscopy Transmission electron microscopy was performed on a JEOL JEM-3200FSC Cryo-TEM, operating at liquid nitrogen temperature. Zero-loss filtered images were obtained at an acceleration voltage of 300 kV. All images were registered digitally by a bottom mounted CCD camera system (Ultrascan 4000, Gatan) combined and processed with a digital imaging processing system (Gatan Digital Micrograph 3.9 for GMS 1.4). Microtomed ultrathin sections were obtained using a LEICA 125 Ultracut microtome. The samples were embedded into epoxy resin prior cutting. UV-Visible spectroscopy UV-Visible spectroscopy was performed on a V-630 UV/Vis Spectrophotometer from Jasco. A clear coat (Proshine, Manhattan, refractive index =1.41) was applied on top of the PVA/NTS film. 1D wide-angle XRD One dimensional wide-angle XRD was performed using an Empyrean setup from PANalytical. An Empyrean Cu x-ray tube LFF HR (line source of 12 × 0.04 mm 2 ) provided CuKα α radiation with λ =1.542 Å at 40 kV voltage and 40 mA current. Bragg Brentano parallel-beam geometry was used. 2D wide-angle XRD Two dimensional wide-angle XRD was performed on a Bruker AXS Nanostar-U Instrument equipped with a microfocus X-ray source (Incoatec ImSCu E025) operating at λ =1.54 Å. A pinhole setup with 750 mm, 400 mm, and 1,000 mm (from source to sample) was used and the sample-to-detector distance was 27 cm. The scattering patterns were corrected for the beam stop and background (Scotch tape) prior to evaluations. The samples were measured at 10–15° (tilt angle) beam inclination with respect to the plane of the films. Intensity distribution profiles in the azimuthal angle were used to calculate the degree of orientation of the nanoclays in the polymer matrix. Degree of orientation is calculated using the following Equation (5): Degree of orientation, where FWHM is the full width at half maximum of the peak in the azimuthal intensity profile. Dynamic light scattering Dynamic light scattering was carried out on an ALV/CGS-3 Compact Goniometer at 23 °C and 90° scattering angle. Tensile mechanical tests Tensile mechanical tests were carried out on a DEBEN minitester equipped with a 20 N load cell. All measurements were conducted at room temperature and specimens were conditioned at required humidity for a minimum of 2 days. The specimen sizes used were in the range of 2 cm × 1.25 mm × 20–30 μm. At least 5 (mostly 9) specimens were tested for each sample at a nominal strain rate of 1 mm min −1 . The slope of the linear region of the stress-strain curves was used to determine the Young’s modulus, E . Water sorption isotherms Water sorption isotherms were performed with a HIDEN ISOCHEMA IGAsorp device at 28 °C in a range of 5−93% RH. Samples ( ca. 9 mg) were exhaustively dried (60 °C) and quickly placed into the machine. The procedure consists of continuous monitoring of the mass of the adsorbed moisture at a particular relative humidity and reaches ca. 95% of the equilibrium mass value before it jumps to the next set %RH. The last 4–5 points of mass values are quasi-static. Oxygen barrier properties Oxygen barrier properties were measured by MOCON (Paul Lippke Handels-GmbH, Neuwied, Germany), using an Ox-tran 2/21 oxygen permeability instrument for PVA/NTS and by Oxygen Permeation Analyser (Systech 8001, Systech Instruments Ltd., U.K.) for PVA/LAP and PVA/SUM (in accordance with ASTM Standard D-3985) at 23 °C and at 80%RH. The active area of measurement was 5 cm 2 . Solid-state 13 C CPMAS NMR Solid-state 13 C CPMAS NMR experiments were performed on a Bruker AV700 NMR spectrometer under cross-polarization magic-angle spinning (CPMAS) condition and spinning at 5 kHz. To improve the efficiency of 1 H– 13 C cross-polarization under MAS a ramp (90/100) contact pulse was applied on the 1 H radio-frequency channel. The duration of the 90° pulse, the dead time of the spectrometer, the dwell time, the contact time, the recycle delay time and the acquisition time were 2 μs, 6 μs, 4 μs, 1.5 ms, 7 s, and 49 ms, respectively. A typical number of 8,192 scans were acquired for each spectrum. All experiments were conducted at 23 °C for PVA/LAP, which was either exhaustively dried or hydrated by D 2 O. How to cite this article: Das, P. et al. Nacre-mimetics with synthetic nanoclays up to ultrahigh aspect ratios. Nat. Commun. 6:5967 doi: 10.1038/ncomms6967 (2015).